A rat RNA-Seq transcriptomic BodyMap across 11 organs and 4 developmental stages The rat has been used extensively as a model for evaluating chemical toxicities and for understanding drug mechanisms. However, its transcriptome across multiple organs, or developmental stages, has not yet been reported. Here we show, as part of the SEQC consortium efforts, a comprehensive rat transcriptomic BodyMap created by performing RNA-Seq on 320 samples from 11 organs of both sexes of juvenile, adolescent, adult and aged Fischer 344 rats. We catalogue the expression profiles of 40,064 genes, 65,167 transcripts, 31,909 alternatively spliced transcript variants and 2,367 non-coding genes/non-coding RNAs (ncRNAs) annotated in AceView. We find that organ-enriched, differentially expressed genes reflect the known organ-specific biological activities. A large number of transcripts show organ-specific, age-dependent or sex-specific differential expression patterns. We create a web-based, open-access rat BodyMap database of expression profiles with crosslinks to other widely used databases, anticipating that it will serve as a primary resource for biomedical research using the rat model. The rat is used extensively by the pharmaceutical, regulatory and academic communities to test drug and chemical toxicities, to evaluate the mechanisms underlying drug effects and to model human diseases. Although several community-wide efforts are preparing a catalogue of genes expressed during normal development of mice [1] , [2] and humans [3] , [4] , such efforts are less advanced for the rat. Furthermore, the rat genome is still incomplete, containing many gaps and missing genes, and the rat transcriptome is not well annotated. Next-generation sequencing technologies have revolutionized genomic research and allow the genome and transcriptome of any organism to be explored without a priori assumptions and with unprecedented throughput [5] , [6] , [7] , [8] , [9] , [10] , [11] . RNA-Seq is able to provide single-nucleotide resolution, strand specificity and short-range connectivity through paired-end sequencing [5] , [8] , [9] , [12] , [13] , [14] . Using RNA-Seq to catalogue the variations in the transcriptome between sexes and over the lifespan of the rat, from birth to old age, can provide insights into disease susceptibility, drug efficacy and safety, and toxicity mechanisms, and could ultimately improve the translation of preclinical findings to humans. Several transcriptomic BodyMap studies have been reported in Drosophila melanogaster [12] , [15] , mouse and human [16] , [17] , [18] , and these studies show large age-dependent variations in gene expression in various organs [19] . In rat, the liver has been examined in detail because of its central role in the metabolism of drugs and xenobiotics [20] , [21] , [22] , [23] . Kwekel et al . [23] found that nearly 3,800 genes in the Fisher 344 rat liver were differentially expressed when evaluated by either age or sex over the life cycle. Such large differences in the transcriptome at various life stages may contribute to age- and/or sex-specific susceptibilities to disease or to adverse reactions to drugs or environmental pollutants. Accounting for these differences may help in developing mechanism-based drug safety assessment and prediction [24] , [25] , as well as in refining environmental risk assessments. Through the US Food and Drug Administration’s sequencing quality control (SEQC) consortium, we use RNA-Seq to comprehensively catalogue transcriptomic profiles across 11 organs and 4 developmental stages (juvenile, adolescence, adult and aged) in both sexes of Fischer 344 rats. To assess inter-animal biological variations, four individual rats are tested per condition. We validate many transcripts that were previously only annotated in AceView [26] based on cDNAs in GenBank and dbEST, including 31,909 alternatively spliced (AS) transcripts and 2,367 spliced non-coding genes/non-coding RNAs (ncRNAs) that were not annotated in RefSeq. This represents the first usage of large amounts of next-generation deep sequence data in rat cross-validated against AceView annotation. We then construct a web-based, open-access rat BodyMap database ( http://pgx.fudan.edu.cn/ratbodymap/index.html ) to catalogue the expression profiles for 40,064 AceView-annotated genes and 65,167 transcripts measured in 320 RNA-Seq libraries, with crosslinks to other widely used databases, including AceView, GenBank, Entrez, Ensembl, RGD, UniProt, Gene Ontology (GO) and Kyoto Encyclopedia of Genes and Genomes. Our study, accompanied by the online database searching capabilities, can serve as a useful resource for both academic biologists and pharmaceutical companies that utilize rats for assessing chemical safety profiles and for studying human diseases. Study design To study the rat transcriptome at single-base resolution, we constructed and sequenced 320 RNA-Seq libraries from 320 RNA samples derived from 16 female and 16 male rats from the Fischer 344 strain. Ten organs were evaluated per rat (adrenal gland, brain, heart, kidney, liver, lung, muscle, spleen, thymus and testis or uterus) at four developmental stages—that is, juvenile (2-weeks old), adolescence (6-weeks old), adult (21-weeks old) and aged (104-weeks old); eight rats (four female and four male rats) were evaluated per developmental stage ( Supplementary Fig. 1 ). To monitor the quality of the RNA-Seq, we added External RNA Control Consortium (ERCC) spike-in controls in an amount equivalent to about 1% of the mRNA in each sample before library construction [27] . RNA-Seq libraries were constructed starting with total RNA using Ribo-Zero kit (Epicentre) for rRNA depletion, combined with Illumina’s TruSeq RNA kit (skipping the Poly(A) + selection step) for each single biological sample, which allowed us to detect both polyadenylated and non-polyadenylated transcripts, including ncRNAs. We generated ~13.2 billion reads of 50-bp single-end RNA-Seq data for this study, corresponding to an average of 40 million sequence reads per sample. Overview of the landscape of the rat transcriptome We mapped the reads to the rat AceView transcriptome [26] , UCSC rn4 genome and ERCC transcripts. On average, 88.5% of the reads were mapped to genomic regions, 41.7% to AceView exons, 8.2% to rRNA and 0.92% to the ERCC transcripts ( Supplementary Fig. 2 ). The pair-wise Pearson correlation coefficient ( R ) between any two of the four biological replicates within each sample group was calculated based on the 40,064 genes, yielding six pair-wise R values per sample group. The mean R value and the s.e. were calculated per group ( n =6), yielding 80 mean R values and 80 s.e. values with a grand mean of 0.9679 and 0.0014 ( n =80), respectively, indicating a high level of measurement consistency among biological replicates ( Supplementary Fig. 3 ). Scatterplots of ERCC log 2 (FPKM) versus log 2 (spike-in concentration) showed an overall linear relationship between RNA-Seq-detected signal and the true concentration of the ERCC spike-in controls, in particular for controls with higher concentrations ( Supplementary Fig. 4a,b and Supplementary Data 1 ). In addition, the average detected expression values of the 92 ERCC controls were similar (log 2 FPKM ~7.2) in 318 of the 320 samples ( Supplementary Fig. 4c ). In general, the expression values of ERCC spike-in controls measured in this study, where an rRNA-depletion protocol (Ribo-Zero) was used for mRNA enrichment, were much closer to the expected values than what was observed using a poly(A)-selection protocol for mRNA enrichment. It was the poly(A)-selection process that introduced the ERCC transcript-specific biases in mRNA enrichment. A combination of quality-control assessment of the sequence data ( Supplementary Figs 3 and 4 ) demonstrated a high level of reproducibility of biological replicates, and the expected behaviour of external spike-in controls ensured that our data are of high quality for follow-up analyses. Consequently, a final data matrix consisting of 40,064 AceView-annotated genes and 65,167 transcripts across all 320 biological samples was generated and used for further analyses as described in the following sections. The mapping pipelines are outlined in Supplementary Fig. 5 . On average, 25,523 (63.7%) of the 40,064 AceView-annotated genes were defined as expressed (FPKM 1) per organ. Differences in the numbers of genes and transcripts expressed were observed among organs, in particular for those only annotated in AceView ( Fig. 1a,b ). For example, 22,995 genes were expressed in the liver, whereas 27,521 were expressed in the lung. Liver and muscle had the lowest numbers of expressed genes in comparison to the other nine organs ( Fig. 1a ). Large numbers of genes (15,894 or 39.7%, Fig. 1a ) and transcripts (27,795 or 42.7%, Fig. 1b ) were expressed in all the 11 organs at all developmental stages and in both sexes, including ‘novel’ genes or transcripts that were annotated only in AceView, but not in RefSeq. 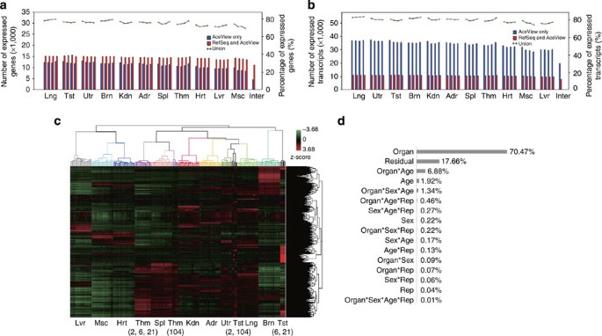Figure 1: Landscape of the rat RNA-Seq transcriptome. Number of expressed genes (a) and transcripts (b) detected per organ across four developmental stages in both males and females (4 biological replicates each). For each panel (a,b), thexaxis indicates organs and developmental stages in either sex, whereas theyaxes (left and right) indicate the numbers of genes or transcripts expressed (× 1,000; left) or the percentages of all annotated genes or transcripts (right) in each organ across four developmental stages in either sex. Red bars represent the number of expressed genes or transcripts (mean±s.e.,N=8; for Tst and UtrN=4) annotated in both RefSeq and AceView, while blue bars represent the additional expressed genes or transcripts (mean±s.e.,N=8; for Tst and UtrN=4) annotated only in AceView. The green lines (unions) represent the number of genes or transcripts expressed per organ and per age in at least one biological replica, male or female (N=8). A gene or transcript was considered expressed if its average expression level in FPKM is1. (c) Hierarchical clustering analysis of gene expression profiles from 320 rat samples with 40,064 genes. (d) Principal variance component analysis (PVCA) of the relative contribution of main effects (organ, age, sex and replicate) and their combinations (asterisk) to total model variance. RefSeq genes are characterized by a gene ID; for RefSeq transcripts, only those well annotated (that is, with ‘NM_’ accessions) were counted. Organs tested are: Adr, adrenal; Brn, brain; Hrt, heart; Kdn, kidney; Lng, lung; Lvr, liver; Msc, skeletal muscle; Spl, spleen; Thm, thymus; Tst, testis; and Utr, uterus; Inter: intersection of genes (a) and transcripts (b) commonly expressed across all 11 organs sampled in this study. The majority of these 15,894 commonly expressed genes (FPKM 1) appear to be primarily involved in basic biological functions—for example, oxidative phosphorylation, GTP–XTP metabolism, cytoskeletal remodelling and the cell cycle ( Supplementary Table 1 ); these genes are referred to as ‘commonly expressed genes’. Figure 1: Landscape of the rat RNA-Seq transcriptome. Number of expressed genes ( a ) and transcripts ( b ) detected per organ across four developmental stages in both males and females (4 biological replicates each). For each panel ( a , b ), the x axis indicates organs and developmental stages in either sex, whereas the y axes (left and right) indicate the numbers of genes or transcripts expressed (× 1,000; left) or the percentages of all annotated genes or transcripts (right) in each organ across four developmental stages in either sex. Red bars represent the number of expressed genes or transcripts (mean±s.e., N =8; for Tst and Utr N =4) annotated in both RefSeq and AceView, while blue bars represent the additional expressed genes or transcripts (mean±s.e., N =8; for Tst and Utr N =4) annotated only in AceView. The green lines (unions) represent the number of genes or transcripts expressed per organ and per age in at least one biological replica, male or female ( N =8). A gene or transcript was considered expressed if its average expression level in FPKM is 1. ( c ) Hierarchical clustering analysis of gene expression profiles from 320 rat samples with 40,064 genes. ( d ) Principal variance component analysis (PVCA) of the relative contribution of main effects (organ, age, sex and replicate) and their combinations (asterisk) to total model variance. RefSeq genes are characterized by a gene ID; for RefSeq transcripts, only those well annotated (that is, with ‘NM_’ accessions) were counted. Organs tested are: Adr, adrenal; Brn, brain; Hrt, heart; Kdn, kidney; Lng, lung; Lvr, liver; Msc, skeletal muscle; Spl, spleen; Thm, thymus; Tst, testis; and Utr, uterus; Inter: intersection of genes ( a ) and transcripts ( b ) commonly expressed across all 11 organs sampled in this study. Full size image To obtain an overview of gene expression profiles of the 320 rat samples, we performed a hierarchical cluster analysis ( Fig. 1c ). This analysis showed a clear separation of the organs by gene expression except for testes and thymus, which are further separated by age group. Testis 2- and 104-week-old differ from testis 6- and 21-week-old, reflecting adolescence and sexual maturity. In contrast, the uterus, even though it mainly contains smooth muscle tissue, was clustered far from both heart and skeletal muscle. The distinct cluster seen in the thymus at 104 weeks reflects the known thymus atrophy in aging animals. Analysis of the sources of variance in our data set by principal variance component analysis showed that organ accounted for 70.47% of the total variance ( Fig. 1d ). All other effects and interactions were less than the residual variance of the model (17.66%). We observed that the sex difference was subtle and only accounted for 0.22% of overall variance in expression profiles. It should be noted that the Y chromosome of the rat has not been sequenced and annotated, explaining the relatively small between-sex differences observed in our data. We, therefore, combined the data from female and male rats for most of our analyses, including those of differentially expressed organ-enriched genes across the four developmental stages. Organ-dependent differentially expressed genes We used a t -test ( P -value 0.05, fold change (FC) 2 or 0.5) to identify genes that were differentially expressed between any two organs. The number of differentially expressed genes (DEGs) was significantly different depending on the pair of organs compared. The overall DEGs between any organ and the other 10 organs over the 4 developmental stages are shown in Fig. 2a . DEGs in the liver and muscle were generally underexpressed compared with the other organs, while DEGs in the brain, testes and lung were generally overexpressed compared with other organs. 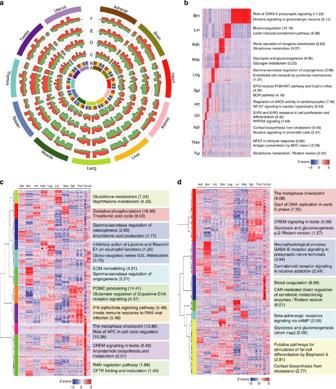Figure 2: Organ- and development-dependent and sex-specific genes. (a) Comparison of relative gene expression between organs. Circos plot illustrating the relative number of DEGs between any two organs (orange, overexpressed; green, underexpressed). Concentric circles from inside to outside represent; A, organ under comparison (colour-coded as described in the outer-most ring); B, the 11 organs being compared with organ A (note no change in DEGs for organ compared with itself); C–F, total number of DEGs, more (orange) or fewer (green) in organ A versus the other organs at weeks 2 (C), 6 (D), 21 (E) or 104 (F). Each bar represents the combination of either four or eight biological replicates for a given organ at the same developmental stage. A gene was considered differentially expressed between two organs if the fold change was2 or0.5 (t-test,P-value0.05). (b) Expression profiles of organ-enriched genes with corresponding significantly and uniquely enriched GeneGo canonical pathway maps. Expression data for 3,413 organ-enriched genes across 320 samples were arranged by organ type (in decreasing order in terms of the number of organ-enriched genes), sex and developmental stage. (c) Development-dependent clusters with significantly enriched GeneGo canonical pathway maps. Development-dependent genes in each organ were identified using a combination of ANOVA with Bonferroni-correctedP0.05 plus a FC2. Hierarchical clustering analysis grouped the development-dependent genes into 10 clusters. (d) Sex-specific clusters with significantly enriched GeneGo canonical pathway maps. The 288 samples (except uterus and testis samples) were separated into 36 groups based on four developmental stages and nine organ types. For any organ at any development stage, genes with a FC2 (or0.5) andP0.05 between female and male were considered sex-specific. Hierarchical clustering analysis grouped the sex-specific genes into six clusters. Expression data wereZ-score standardized (mean zero and s.d. of one) per gene. Ontology terms of enriched GeneGo canonical pathway maps were listed next to each organ type (b) or cluster (c,d) on the right along with –log10(FDRq-value) in the parentheses. Organs tested are: Adr, adrenal; Brn, brain; Hrt, heart; Kdn, kidney; Lng, lung; Lvr, liver; Msc, skeletal muscle; Spl, spleen; Thm, thymus; Tst, testis; and Utr, uterus. Figure 2: Organ- and development-dependent and sex-specific genes. ( a ) Comparison of relative gene expression between organs. Circos plot illustrating the relative number of DEGs between any two organs (orange, overexpressed; green, underexpressed). Concentric circles from inside to outside represent; A, organ under comparison (colour-coded as described in the outer-most ring); B, the 11 organs being compared with organ A (note no change in DEGs for organ compared with itself); C–F, total number of DEGs, more (orange) or fewer (green) in organ A versus the other organs at weeks 2 (C), 6 (D), 21 (E) or 104 (F). Each bar represents the combination of either four or eight biological replicates for a given organ at the same developmental stage. A gene was considered differentially expressed between two organs if the fold change was 2 or 0.5 ( t -test, P -value 0.05). ( b ) Expression profiles of organ-enriched genes with corresponding significantly and uniquely enriched GeneGo canonical pathway maps. Expression data for 3,413 organ-enriched genes across 320 samples were arranged by organ type (in decreasing order in terms of the number of organ-enriched genes), sex and developmental stage. ( c ) Development-dependent clusters with significantly enriched GeneGo canonical pathway maps. Development-dependent genes in each organ were identified using a combination of ANOVA with Bonferroni-corrected P 0.05 plus a FC 2. Hierarchical clustering analysis grouped the development-dependent genes into 10 clusters. ( d ) Sex-specific clusters with significantly enriched GeneGo canonical pathway maps. The 288 samples (except uterus and testis samples) were separated into 36 groups based on four developmental stages and nine organ types. For any organ at any development stage, genes with a FC 2 (or 0.5) and P 0.05 between female and male were considered sex-specific. Hierarchical clustering analysis grouped the sex-specific genes into six clusters. Expression data were Z- score standardized (mean zero and s.d. of one) per gene. Ontology terms of enriched GeneGo canonical pathway maps were listed next to each organ type ( b ) or cluster ( c , d ) on the right along with –log 10 (FDR q- value) in the parentheses. Organs tested are: Adr, adrenal; Brn, brain; Hrt, heart; Kdn, kidney; Lng, lung; Lvr, liver; Msc, skeletal muscle; Spl, spleen; Thm, thymus; Tst, testis; and Utr, uterus. Full size image We looked to identify organ-enriched genes that were highly expressed and relatively specific to each organ. To identify organ-enriched genes during development ( Supplementary Fig. 6 ), we used a t -test with a Bonferroni-corrected P -value 0.05 to generate a list of organ-enriched genes at increasing FC cutoff values (that is, 2, 4, 8, 16, 32, 64, 128 and 256). When a FC of 2 was used, we identified 3,413 organ-enriched AceView genes ( Supplementary Table 2 ), 2,052 (60.1%) of which were annotated in RefSeq and the remaining 1,361 (39.9%) annotated only in AceView. Of these organ-enriched genes, 1,401 (41.0%) were detected specifically in the brain, 454 (13.3%) specifically in the liver and 386 (11.3%) specifically in the kidney ( Supplementary Table 2 ). The numbers of organ-enriched genes identified in the other eight organs ranged from 25 to 306. Organ-enriched genes reflect organ biological functions We conducted GO enrichment analysis of organ-enriched genes in each organ type that were annotated in RefSeq ( n =2,052; Fig. 2b ). Supplementary Data 2 contain a list of all pathways that were significantly enriched ( P 0.05, hypergeometric test, Benjamini–Hochberg FDR-adjusted P -value) and unique to each organ. In general, the GO enrichment and the selection and ranking of the pathways based on organ-enriched genes were highly consistent with the biological functional activities of the organ for which the genes were enriched. 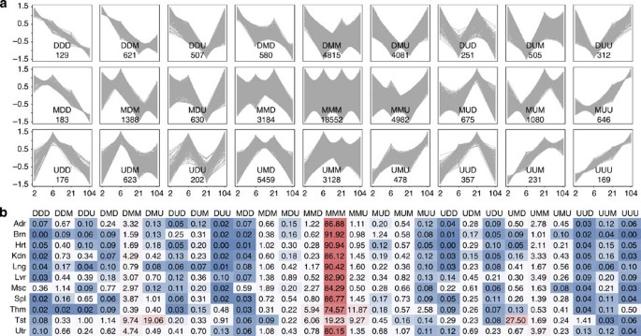Figure 3: Development-dependent patterns of rat gene expression. (a) Differentially expressed genes were determined based on a combination of ANOVA with the Bonferroni-correctedP-value0.05 and FC2 (or0.5) between the four developmental stages. For each organ, data from two sequential developmental stages were compared, with the younger developmental stage used as the denominator. Genes were grouped into Up (U; ‘upregulated’ based on FC2), Down (D; ‘downregulated’ based on FC0.5), or Maintain (M; ‘no change’ based on 0.5<FC<2). Shown here are the 27 possible combinatorial patterns. Thexaxis depicts time point (in weeks) and theyaxis depicts fold change. The number shown in each box (for example, 129 genes for pattern DDD) was derived based on the number of genes, across all 11 organs—where each gene was counted only once regardless of how many organs shared that same pattern. (b) The percentage of genes within each pattern per organ exhibiting specific development-dependent expression patterns. The numbers in the table are colour-coded; red indicates a relatively large percentage of genes with that expression pattern and blue represents a relatively small percentage of genes with that pattern. Organs tested are: Adr, adrenal; Brn, brain; Hrt, heart; Kdn, kidney; Lng, lung; Lvr, liver; Msc, skeletal muscle; Spl, spleen; Thm, thymus; Tst, testis; and Utr, uterus. For example, brain-enriched genes were associated with neurophysiological processes including dopamine and GABA signalling, whereas heart-enriched genes were associated with muscle contraction, signal transduction and regulation of cardiac hypertrophy ( Supplementary Table 3 ). Examples of pathways defined by the organ-enriched genes are shown for the brain (role of CDK5 in presynaptic signalling, Supplementary Fig. 7 ), liver (bile acid biosynthesis, Supplementary Fig. 8 ) and kidney (renal secretion of organic electrolytes, Supplementary Fig. 9 ). Development-dependent genes To evaluate development-dependent differential gene expression in various organs, we used an analysis of variance (ANOVA) model and applied FC 2 (or 0.5) plus a Bonferroni-adjusted P -value 0.05. Overall, we identified 18,640 genes differentially expressed during development in at least one of the 11 organs, of which 10,572 were annotated in both RefSeq and AceView; the remaining 8,068 were only annotated in AceView. 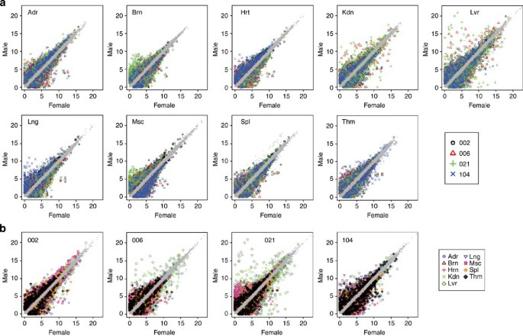Figure 4: Sex differences of rat transcriptomic profiles. Gene expression values, expressed as log2FPKM, for male (yaxis) and female (xaxis) rats are depicted in the scatter plots. These plots show gene expression profiles between female and male rats in nine organs (a) and four developmental stages (b) using pooled data from either all four stages (a) or all organs for a given stage (b). Non-DEGs form the centre line (in grey), while DEGs are coloured and occur above and below the centre line. 002=2 weeks; 006=6 weeks; 021=21 weeks; 104=104 weeks. Organs tested are: Adr, adrenal; Brn, brain; Hrt, heart; Kdn, kidney; Lng, lung; Lvr, liver; Msc, skeletal muscle; Spl, spleen; and Thm, thymus. The number of development-dependent genes varied by organ, from 2,211 in the brain to 16,186 in the testis ( Supplementary Table 4 ). As expected, the greatest differential gene expression was observed when juvenile 2-week-old rats were compared with older rats. Moreover, a large number of genes were differentially expressed in the testis across ages, as seen in a comparison with sexually mature 6- and 21-week-old rats with 2- and 104-week-old rats ( Supplementary Table 4 ), which have young and atrophying testes, respectively. Major known functions of the 10,572 development-dependent DEGs annotated in RefSeq included protein folding and maturation, cell cycle, cell adhesion, immune response, glutathione metabolism and transcription ( Fig. 2c and Supplementary Data 3 ). Development-dependent gene expression patterns To evaluate the time course and development-dependent transcriptomic activities across the life cycle of the rat, we performed a time course differential gene expression analysis by comparing any two adjacent developmental stages, using the younger developmental stage group as the denominator (see Online Methods) for each of the 11 organs. There were 27 possible patterns (three change points during development, or 3 3 possibilities), including those that increased across all developmental stage boundaries, termed ‘up-up-up’ (UUU); those that were similar across all boundaries, termed ‘maintain-maintain-maintain’ (MMM); and those that decreased across all boundaries, termed ‘decrease-decrease-decrease’ (DDD). Genes were non-randomly represented across all patterns. The overall development-dependent patterns across all organs are shown in Fig. 3a . Relatively few genes continuously increased (UUU) or decreased (DDD) in expression during aging, the vast majority of genes remained unchanged over the lifespan (over 74% for any organ except for the testis) ( Fig. 3b ). However, the onset of adolescence and adulthood triggers significant changes in genes (UMM or DMM) as well as the onset of old age (MMD or MMU) ( Fig. 3 ). Figure 3: Development-dependent patterns of rat gene expression. ( a ) Differentially expressed genes were determined based on a combination of ANOVA with the Bonferroni-corrected P -value 0.05 and FC 2 (or 0.5) between the four developmental stages. For each organ, data from two sequential developmental stages were compared, with the younger developmental stage used as the denominator. Genes were grouped into Up (U; ‘upregulated’ based on FC 2), Down (D; ‘downregulated’ based on FC 0.5), or Maintain (M; ‘no change’ based on 0.5<FC<2). Shown here are the 27 possible combinatorial patterns. The x axis depicts time point (in weeks) and the y axis depicts fold change. The number shown in each box (for example, 129 genes for pattern DDD) was derived based on the number of genes, across all 11 organs—where each gene was counted only once regardless of how many organs shared that same pattern. ( b ) The percentage of genes within each pattern per organ exhibiting specific development-dependent expression patterns. The numbers in the table are colour-coded; red indicates a relatively large percentage of genes with that expression pattern and blue represents a relatively small percentage of genes with that pattern. Organs tested are: Adr, adrenal; Brn, brain; Hrt, heart; Kdn, kidney; Lng, lung; Lvr, liver; Msc, skeletal muscle; Spl, spleen; Thm, thymus; Tst, testis; and Utr, uterus. Full size image Sex-specific DEGs Even though they represented a small proportion of overall variation in gene expression, differential gene expression profiles between female and male rats for all nine non-sex organs were examined at all four developmental stages ( Figs 4a,b , and Supplementary Fig. 10 ). A number of genes were significantly different between male and female rats, particularly in the liver, muscle and kidney, and to a lesser extent in the spleen and brain. 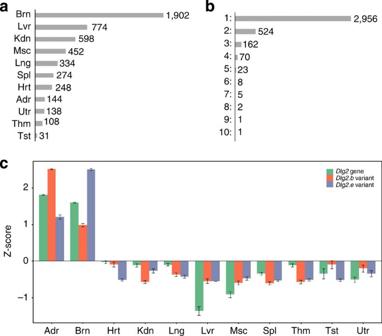Figure 5: Organ-enriched alternatively spliced transcript expression. (a) Numbers of organ-specific transcript variants for both female and male rats across the four developmental stages. A transcript was considered an organ-specific alternatively spliced variant if it had an FC2 plus a Bonferroni-correctedP-value0.05 when compared with its expression in other organs across the four developmental stages. (b) Organ-specific transcript variant abundance. Distribution of genes (on the right) with a given number of variants (1 thru 10). (c) Organ-specific transcript variant expression forDlg2. Theyaxis represents normalized (Mean=0 and s.d.=1) expression profile (mean±s.e.,N=32 (or 16 for Tst and Utr))Z-score and thexaxis representsDlg2gene (green),Dlg2.bvariant (orange) andDlg2.evariant (blue) expression in each organ. Organs tested are: Adr, adrenal; Brn, brain; Hrt, heart; Kdn, kidney; Lng, lung; Lvr, liver; Msc, skeletal muscle; Spl, spleen; Thm, thymus; Tst, testis; and Utr, uterus. Most DEGs were found at 21 weeks, in adults ( Supplementary Table 5 ). More notable were, at 6 weeks, the 2,230 female-dominant genes (sexually dimorphic expression with higher expression in female) compared with 1,668 male-dominant genes (sexually dimorphic expression with higher expression in male). Female-dominant genes were outnumbered by male-dominant genes at all other ages (female versus male: 1,921 versus 3,409 for week 2; 2,769 versus 2,945 for week 21; and 2,116 versus 2,571 for week 104). More genes showed sex-specific expression in the liver and kidney in week 21 with large FCs ( Fig. 4a,b , and Supplementary Table 5 ). Genes involved in metabolism, particularly cytochrome P450s, are also known to be differentially expressed between the sexes. We found P450 differences to be variable; however, expression levels of Cyp1a1 , Cyp1a2 , Cyp2c7 , Cyp3a9 and Cyp26a1 were higher in the female liver, predominantly at sexual maturity, whereas Cyp2a2 , Cyp2c , Cyp3a2 and Cyp3a18 were expressed higher in the male liver (data not shown). Major known functions of the 6,677 sex-specific DEGs annotated in RefSeq included cell cycle, blood coagulation and CREM signalling in the testis and GABA-B receptor signalling in presynaptic nerve terminals ( Fig. 2d and Supplementary Data 4 ). Figure 4: Sex differences of rat transcriptomic profiles. Gene expression values, expressed as log 2 FPKM, for male ( y axis) and female ( x axis) rats are depicted in the scatter plots. These plots show gene expression profiles between female and male rats in nine organs ( a ) and four developmental stages ( b ) using pooled data from either all four stages ( a ) or all organs for a given stage ( b ). Non-DEGs form the centre line (in grey), while DEGs are coloured and occur above and below the centre line. 002=2 weeks; 006=6 weeks; 021=21 weeks; 104=104 weeks. Organs tested are: Adr, adrenal; Brn, brain; Hrt, heart; Kdn, kidney; Lng, lung; Lvr, liver; Msc, skeletal muscle; Spl, spleen; and Thm, thymus. Full size image Using a gene with many different alternatively spliced variants as an illustration, we also explored the organ-dependent and sex-specific differential isoform expression of Ugt1a1 (UDP glucuronosyltransferase 1 family, polypeptide A1), an enzyme playing an essential role in the detoxification of xenobiotics and endogenous compounds by conjugating bilirubin with glucuronic acid [28] , [29] , [30] . Twelve Ugt1a1 isoforms were annotated for rat in AceView, two of which ( Ugt1a1 g and h ) showed organ-dependent differential expression between female and male rats. Ugt1a1 h was expressed significantly higher in female liver, while Ugt1a1 g was more highly expressed in the male adrenal gland and lung ( Supplementary Fig. 11 ). The Ugt1a1 gene itself, as well as its other 10 isoforms (data not shown), did not show any sex-specific differential expression. Alternative splicing and organ-specific isoform expression On the basis of the cDNA sequences deposited in NCBI GenBank and dbEST databases, 2,430 novel spliced non-coding genes have been annotated in AceView. Among them, 2,367 non-coding genes were cross-validated with the data set from the current study ( Supplementary Data 5 ). We also cross-validated 31,909 alternatively spliced transcripts ( Supplementary Data 6 ) only annotated in AceView. Both of these tables are linked to AceView. We further measured and mapped the expression level of these alternatively spliced transcripts and non-coding genes/ncRNAs across the 11 organs in our rat BodyMap database. Of the 2,367 spliced non-coding genes, 326 were expressed in all organs across the four developmental stages ( Supplementary Fig. 12a ), whereas 139 displayed organ-enriched expression, with 44 specifically expressed in the brain ( Supplementary Fig. 12b ). We found that soyshee , one of the spliced non-coding genes/ncRNAs in AceView, was most highly expressed in the liver with somewhat lesser expression in the testis (6 and 21 weeks, Supplementary Fig. 13 ). We also examined the expression of all alternatively spliced transcripts (including those annotated in RefSeq). The brain contained the vast majority of organ-enriched transcript variants (1,902) followed by the liver (774), kidney (598) and muscle (452) ( Fig. 5a ). The number of organ-enriched transcript variants per gene varied from 1 to 10, with 2,956 genes having one variant, 23 genes having five variants and one gene having 10 variants defined as organ-enriched ( Fig. 5b ). Most of the organ-enriched transcript variants showed the same expression pattern as the gene itself. However, some organ-enriched transcript variants showed a different, organ-dependent expression pattern, such as Dlg2 (disks large homologue 2, Fig. 5c ). In addition to Dlg2 variant a , which is annotated in RefSeq, five additional Dlg2 variants (named Dlg2.b, c, d, e and f ) were annotated in AceView. Dlg2.b was highly enriched in the adrenal gland, whereas Dlg2 . e . was enriched in the brain. Another gene that showed organ-specific differential variant expression was Pecr (peroxisomal trans-2-enoyl-CoA reductase), coding for an enzyme involved in fatty acid elongation [31] , [32] . Four transcript variants (named a , b , c and d ) were annotated in AceView. Our data demonstrated that, while the Pecr gene, as well as its variants a and d , showed a similar expression profile and were highly enriched in the liver, Pecr.c was expressed almost exclusively in the kidney ( Supplementary Fig. 14 ). Figure 5: Organ-enriched alternatively spliced transcript expression. ( a ) Numbers of organ-specific transcript variants for both female and male rats across the four developmental stages. A transcript was considered an organ-specific alternatively spliced variant if it had an FC 2 plus a Bonferroni-corrected P -value 0.05 when compared with its expression in other organs across the four developmental stages. ( b ) Organ-specific transcript variant abundance. Distribution of genes (on the right) with a given number of variants (1 thru 10). ( c ) Organ-specific transcript variant expression for Dlg2 . The y axis represents normalized (Mean=0 and s.d.=1) expression profile (mean±s.e., N =32 (or 16 for Tst and Utr)) Z -score and the x axis represents Dlg2 gene (green), Dlg2.b variant (orange) and Dlg2 . e variant (blue) expression in each organ. Organs tested are: Adr, adrenal; Brn, brain; Hrt, heart; Kdn, kidney; Lng, lung; Lvr, liver; Msc, skeletal muscle; Spl, spleen; Thm, thymus; Tst, testis; and Utr, uterus. Full size image Transcriptional expression profiles can also serve as an important resource for developing a functional understanding of regulation of splicing events and selection of alternative promoters and polyadenylation sites [33] , [34] , [35] . For example, troponin Tnni1.c and Tnni1.d variants were both annotated in AceView as encoding the same isoform of troponin 1, skeletal, slow 1, but differ by AS affecting the 3′ untranslated region (UTR) and alternative polyadenylation (APA) site selection. Illustration of the AS/APA events and expression patterns in three organs of 6-week-old female rats are shown ( Fig. 6a ). As expected for troponin protein-coding transcripts, neither Tnni1.c nor Tnni1.d were expressed in the brain, but both were highly expressed in the muscle, where expression of Tnni1.d was 94% higher than that of Tnni1.c. Interestingly, only Tnni1.d , which is an AceView-only transcript, was detectable in the thymus (proportion value =0.994, see Online Methods). The underlying biological mechanism of the organ-dependent expression of Tnni1.c and Tnni1.d warrants further investigation. 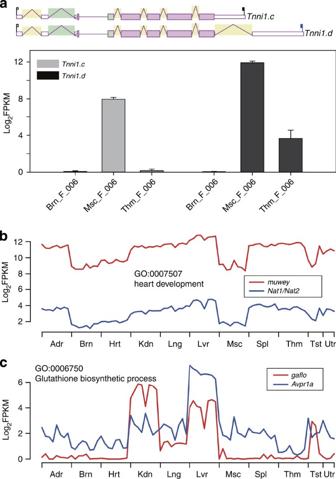Figure 6: Alternative polyadenylation variants. (a) An example of alternative splicing and polyadenylation. The upper panel of (a) shows the alternate variants c and d of geneTnni1, both encoding the same protein isoform of troponin 1, skeletal, slow 1. A white thin box represents a UTR, whereas pink means a protein-coding region, and the solid black and blue flags in the 3′-UTRs represent the canonical and non-canonical poly-A signals used for polyadenylation, respectively. The expression levels of these two transcripts in brain (Brn), skeletal muscle (Msc) and thymus (Thm) of female (F) rats at week 6 (006) are shown in barplots, with error bars representing the s.e. of expression values (log2FPKM) across the four biological replicates. (b,c) Two examples of co-expression-based functional prediction. Each example includes the expression values (log2FPKM) of two genes, one with annotated functions (blue) and the other without (red) across the 80 sample groups ordered first by organ, then by sex (except for testis and uterus) and at last by age. The GO term shown for each example represents the function of the annotated gene (Nat1/Nat2orAvpr1a) and is the predicted function of the corresponding non-annotated gene (spliced non-coding genemuweyor spliced coding genegaflo). Organs tested are: Adr, adrenal; Brn, brain; Hrt, heart; Kdn, kidney; Lng, lung; Lvr, liver; Msc, skeletal muscle; Spl, spleen; Thm, thymus; Tst, testis; and Utr, uterus. Figure 6: Alternative polyadenylation variants. ( a ) An example of alternative splicing and polyadenylation. The upper panel of ( a ) shows the alternate variants c and d of gene Tnni1 , both encoding the same protein isoform of troponin 1, skeletal, slow 1. A white thin box represents a UTR, whereas pink means a protein-coding region, and the solid black and blue flags in the 3′-UTRs represent the canonical and non-canonical poly-A signals used for polyadenylation, respectively. The expression levels of these two transcripts in brain (Brn), skeletal muscle (Msc) and thymus (Thm) of female (F) rats at week 6 (006) are shown in barplots, with error bars representing the s.e. of expression values (log 2 FPKM) across the four biological replicates. ( b , c ) Two examples of co-expression-based functional prediction. Each example includes the expression values (log 2 FPKM) of two genes, one with annotated functions (blue) and the other without (red) across the 80 sample groups ordered first by organ, then by sex (except for testis and uterus) and at last by age. The GO term shown for each example represents the function of the annotated gene ( Nat1 / Nat2 or Avpr1a ) and is the predicted function of the corresponding non-annotated gene (spliced non-coding gene muwey or spliced coding gene gaflo ). Organs tested are: Adr, adrenal; Brn, brain; Hrt, heart; Kdn, kidney; Lng, lung; Lvr, liver; Msc, skeletal muscle; Spl, spleen; Thm, thymus; Tst, testis; and Utr, uterus. Full size image For genes without any clear function description in AceView, their co-expression patterns across the 320 RNA samples with genes of known functions under the same GO term has the potential to provide an indication of their functions based on the ‘guilty by association’ principle (see Online Methods). Two examples of functional inference are shown in Fig. 6b,c . The gene muwey was annotated in AceView with one potential non-coding transcript. Our RNA-Seq data showed that the trend of expression profile of muwey across the 320 rat RNA samples was highly similar to that of the gene Nat1/Nat2 , which is a member of the GO:0007507 (heart development) group; thus, the function of muwey may also be associated with heart development. However, we note that the absolute expression level of muwey was much higher than that of Nat1 / Nat2 . Similarly, the AceView-only gene gaflo may be related to the glutathione biosynthetic process because its expression profile was similar to that of Avpr1a , a member of the GO:0006750 group (glutathione biosynthetic process). We investigated the transcriptome of the Fischer 344 rat by constructing a rat RNA-Seq transcriptomic BodyMap including 11 organs, from both sexes, at 4 developmental stages from juvenile to old age. Although many genes showed organ-specific differential expression across the lifespan, thousands of genes were commonly expressed across all organs and 4 developmental stages. Interestingly, genes that were commonly expressed in all organs were more likely to be annotated in RefSeq than in AceView, while genes that were enriched in organs were increasingly represented in AceView. RefSeq contains well-studied genes expressed at high levels, mostly the conserved coding genes. AceView [26] is a more comprehensive annotation based on cDNAs and is more likely to contain novel or uncommon genes. We found that organ-enriched genes are well correlated with the biological functions of each organ. For example, brain-enriched genes were active in pathways related to a variety of neurophysiological processes, including dopamine signalling, CDK5 signalling and GABA signalling. The pathway enrichment pattern for liver-enriched genes was very different from that for the brain and included various metabolic processes such as fatty acid oxidation and bile acid biosynthesis, whereas thymus-enriched genes were associated with various immune-related processes and signalling pathways. In contrast, genes defined as commonly expressed across all organs tended to be enriched in non-organ-specific pathways such as oxidative phosphorylation, GTP–XTP metabolism and cytoskeleton remodelling. Sex-specific and organ-dependent differential gene expression was also intriguing [22] , [23] . We catalogued many genes, along with their alternatively spliced isoforms, that demonstrated organ-dependent and sex-specific expression, such as Ugt1a1 , an essential enzyme responsible for conjugation and elimination of bilirubin. We found that Ugt1a1 h was expressed significantly higher in the female liver, whereas Ugt1a1 g was more abundantly expressed in the male adrenal gland and lung. Further functional investigation into the sex-dependent and organ-specific differential isoform expression of Ugt1a1 g and h is needed. Alternative splicing of genes is a critical mechanism in organ development during organ formation in complex organisms [3] , [4] . Abnormal organ-specific expression of isoforms may cause human diseases [35] . We catalogued and determined the expression of 31,909 AceView-only alternatively spliced transcripts in rat. Some genes, such as Dlg2 . b and Dlg2 . e , displayed differential organ-specific expression of splice variants and are enriched in the adrenal gland and brain, respectively. Over the last decade, evidence from numerous experiments indicates that not only the protein-coding region but also the non-coding region of the genome regulates the complexity of organisms as well as developmental processes [36] . Using a combination of computational analysis on human and mammalian cDNAs/ESTs and extensive manual curation, the ENCODE consortium has catalogued 9,640 lncRNA loci representing 15,512 transcripts in humans [3] , [4] , [36] . This is to be compared with the AceView human annotation that catalogues 11,122 spliced non-coding genes represented by 21,710 transcripts [26] . However, a similar investigation in rat is limited by the scarcity of rat cDNA sequences in GenBank. Here we catalogued 2,367 novel spliced non-coding genes/ncRNAs in rat. Further functional characterization of these non-coding genes/ncRNAs will be important in maximizing the utility of the rat model for drug safety and efficacy evaluation. Our RNA-Seq data set, which is readily accessible through our web-based database search system, consists of a diverse set of 320 samples from multiple organs of both male and female rats across the life cycle. It can be used to better annotate the rat transcriptome and to identify novel transcripts and novel genes. The expression profile of a novel transcript or gene across the 320 samples could be used as a fingerprint for inferring its normal biological function by comparing it with expression profiles of other transcripts or genes of known functions (for example, Figs. 6b,c ). In addition, organ- and sex-specific expression patterns could be utilized for studying the pharmacological and toxicological effects of drugs that might be organ- or sex-dependent. Furthermore, the rat gene expression BodyMap reported here could be used as a basis for cross-species comparison, facilitating better translation of preclinical animal safety data to human health. In summary, we have generated a comprehensive rat RNA-Seq transcriptomic BodyMap encompassing 11 organs across 4 developmental stages from juvenile to old age for both sexes. As a unique public resource for gene expression, this BodyMap is expected to provide a comprehensive platform for biomedical research by enabling increased understanding of human diseases and improved assessment of drug efficacy and toxicity with the rat model [24] , [25] . Methods and any associated references are available in the online version of the paper. Animals and organ collection Female and male Fischer 344 rats (pair-housed under standard conditions) from the National Center for Toxicological Research of the US Food and Drug Administration animal-breeding colony were euthanized by carbon dioxide asphyxiation at 2, 6, 21 and 104 week-of-age as previously described [23] . Organs (liver, heart, kidney, brain, lung, gastrocnemius muscle, spleen, thymus, adrenal gland, uterus (females), and testes (males)) from 2-week-old (juvenile), 6-week-old (adolescence), 21-week-old (adult) and 104-week-old (aged) rats were used in this study ( Supplementary Fig. 1 ). At necropsy, whole organs were removed, quick-frozen in liquid N 2 and stored at −80 °C for RNA extraction. Organs were harvested from four male and four female rats at each of the four developmental stages. This study had ethical and scientific approval from the National Center for Toxicological Research Institutional Animal Care and Use Committee. The rats were housed and euthanized according to the NIH and institutional guidelines. RNA isolation Each whole organ was individually ground (mortar and pestle, under continuous liquid N 2 chilling) into a fine powder before RNA extraction, with the exception of the liver, spleen and gastrocnemius muscle for which ~100 mg was ground. Ground organ tissue was stored at −80 °C. Total RNA was extracted from ~30 mg of ground tissue by using the miRNeasy Mini Kit (Qiagen) according to the manufacturer’s protocol, including treatment with DNase. RNAs longer than 18 nucleotides were recovered with this method. RNA quality was evaluated with an Agilent 2100 Bioanalyzer (Agilent Technologies). All RNA samples had RNA integrity numbers (RINs) greater than 7.5, except for the eight spleen samples from rats of both sexes at 2 weeks-of-age (RIN: 2.2–5.1). Excluding these spleen samples, the average RIN was 9.2 for the other 312 RNA samples. Construction of rRNA-depleted RNA-Seq libraries We used an rRNA depletion protocol coupled with the Illumina TruSeq RNA-Seq library protocol to construct the rat Bodymap RNA-Seq libraries. For each of the 320 RNA samples, one single RNA-Seq library was constructed. Total RNA (1 μg) spiked with 2 μl 1:100 diluted ERCC RNA spike-in control mix 1 or mix 2 (Life Technologies) was depleted of rRNA with the Ribo-Zero Nonmagnetic Kit (Epicentre). The rRNA-depleted RNA was purified using the RNA Clean & Concentrator Column (Zymo Research), which recovered all rRNA-depleted RNA, including small RNA (>17 nt). We then used the TruSeq RNA Sample Preparation Kit (Illumina) but skipped the Poly(A) + selection step during library construction. The rRNA-depleted RNA was fragmented, followed by first and second strand cDNA synthesis. The cDNA was subject to end repair, adenylation of 3′ ends and adapter ligation. We used one of 12 unique indices in each randomized sample (for multiplexing). cDNA samples were purified using AMPure XP beads (Beckman Coulter) and then used in 15 cycles of PCR amplification (ABI GeneAmp PCR system 9700). The cDNA library quality and size distribution were checked using an Agilent Bioanalyzer and DNA 1000 chip. Library fragment sizes were between 200 and 500 bp, with a peak at ~260 bp. All libraries were quantified with a Qubit 2.0 Fluorometer (Life Technologies) and stored in non-sticky Eppendorf tubes (Life Technologies) at −20 °C. RNA-Seq library sequencing RNA-Seq libraries were sequenced using Illumina’s TruSeq Cluster V3 flow cells and TruSeq SBS Kit V3 (Illumina). The 320 rat Bodymap libraries were clustered using TruSeq V3 flow cells, with 10 libraries of different indices in each lane at a concentration of ~8.6 pM, and sequenced (50 bp single end read) on an Illumina HiSeq 2000 by Expression Analysis Inc. Ten different RNA-Seq libraries (biological samples, randomized) were pooled together in equal amount and loaded in one single lane on two different flow cells for sequencing, which would give two technical replicates from each biological sample. Reads from the two technical replicates of the same RNA sample were combined together to represent sequencing readouts for each biological sample. Read mapping and quantification Data were first trimmed using Trimmomatic [38] . We used the rat transcriptome from AceView [26] v08, which includes 40,064 unique genes, as reference (downloaded from ftp://ftp.ncbi.nih.gov/repository/acedb/ncbi_4_Sep08.rat.genes ). In addition, the rat genome UCSC rn4, downloaded from iGenome (ftp://igenome:G3nom3s4u@ussd-ftp.illumina.com/Rattus_norvegicus/UCSC/rn4/Rattus_norvegicus_UCSC_rn4.tar.gz), was used as a reference genome. Reads were aligned to the rat reference genome and AceView transcriptome with TopHat v2.0.4 (ref. 37 ), allowing a maximum of two mismatches in the alignment. The default parameter settings were used. Alignment results were then processed using Cufflinks v2.0.2 (ref. 39 ) for gene and transcript quantification ( Supplementary Fig. 5 ). ERCC transcript sequences were obtained from NCBI (Accession codes are listed in Supplementary Table 6 ). Reads that were unable to align to the rat genome were converted to fastq format using bam2fastq ( http://www.hudsonalpha.org/gsl/information/software/bam2fastq ) for ERCC mapping and calculation. Reads were then mapped to ERCC transcripts and quantified using TopHat v2.0.4 and Cufflinks v2.0.2 with the same parameters described above. For samples with two to three technical replicates, average FPKM (fragment per kilobase per million mapped reads) values were used. To avoid infinite values, a value of 1 was added to the FPKM value of each gene before log 2 transformation. AceView transcriptome annotation AceView gene models integrate 734,000 rat cDNA sequences available in GenBank in addition to the RefSeq sequences. Although the public cDNA contribution of rat only contains 1/10 the coverage of human or 1/4 of mouse, it nevertheless enriches the rat genes without introducing a bias in favour of coding versus non-coding sequences. There were 40,064 genes and 65,167 transcripts annotated in AceView, with 45,126 alternatively spliced variants having full experimental support. Among these AceView genes and transcripts, 19,449 genes and 14,217 transcripts were annotated as RefSeq (NM_) genes and transcripts. Analysis of transcriptomic gene expression profiles In our analyses, a gene was considered to be expressed in a sample if its expression value in FPKM was equal or greater than 1 in the sample. Furthermore, a gene was considered ‘commonly’ expressed if it was expressed in all organs, at all developmental stages, and in both sexes, and if its expression in FPKM was more than 1 in three aspects: mean for each organ, mean at each time point for each organ and mean for each sex at each time point in each organ. Hierarchical clustering analysis (HCA) was performed using Ward linkage based on a distance matrix of the Pearson correlation of the samples, using R package [40] . In this study, DEGs were identified as recommended and reported in our previous MAQC publications, with a FC ranking in expression value of FPKM and a nonstringent P -value cutoff of 0.05 in log-transformed expression value (log 2 FPKM) [41] , [42] . Other analyses, such as Pearson correlation, Student’s t -test, principal component analysis and HCA, were performed using functions in R as follows: ‘cor’, ‘t.test’, ‘prcomp’ in the ‘stats’ package, and heatmap.2 in ‘gplots’ package. Circos [43] was used to draw the graphs of the number of DEGs identified among organs. Principal variance component analysis (PVCA) was used to calculate the relative contributions of main effects (organ, age, sex and replicate) and their combinations in (asterisk) to total model variance. The quantitative sources of variance were estimated using PVCA within JMP Genomics 6.0 (SAS Institute Inc., Cary, NC, USA). PVCA integrates two methods to estimate the variance components: principal component analysis (PCA) and variance component analysis. Principal component analysis finds low-dimensional linear combinations of data with maximal variability, whereas variance component analysis attributes and partitions variability into known sources via a classical random effects model. Organ-enriched development-dependent and sex-specific genes Organ-enriched genes were identified using FCs of 2, 4, 8, 16, 32, 64, 128 and 256, with a Bonferroni-corrected P 0.05 across four developmental stages ( Supplementary Fig. 6 ). Age-dependent genes were defined as genes whose expression values differed significantly among the four development stages. Time course DEG analysis was performed by comparing different developmental stages for each organ. To identify development-dependent genes in each organ, we used a combination of ANOVA with Bonferroni-corrected P 0.05 plus a FC 2 to select genes that were differentially expressed between developmental stages. Sex-specific genes were examined between female and male rats for all nine non-sex organs at all four developmental stages. All 288 samples (except uterus and testis samples) were separated into 36 groups based on four developmental stages and nine organ types. FC and t -test P -value were calculated between female and male in each organ across four time points ( Supplementary Fig. 10 ). For any organ at any development stage, genes with a FC 2 (or 0.5) and P 0.05 were considered to be sex-specific. Analysis of development-dependent gene expression patterns Development-dependent genes were identified as described previously. In each organ, comparisons were made between two adjacent developmental stages, with the younger developmental stage as denominator—that is, 6- veusus 2-weeks old, 21- versus 6-weeks old and 104- versus 21-weeks old. A gene with FC 2 was grouped into the ‘up’ pattern and considered as upregulated during that developmental stage bracket. A gene with FC 0.5 was grouped into ‘decrease’, and the remaining genes were grouped into ‘maintain’. Thus, in each organ, a gene was grouped to 1 out of 27 patterns, ranging from up-up-up (UUU), maintain-maintain-maintain (MMM), to decrease-decrease-decrease (DDD). Pathway analysis To identify pathways and biological processes of the organ-enriched genes, sex-specific clusters or development-dependent clusters of genes, the lists of genes (both up- and downregulated) were evaluated with protein groupings from the MetaCore canonical pathway maps ontology (Thomson Reuters). This ontology represents images of three to six signalling pathways that describe a biological mechanism. Signalling pathways are linear multistep chains of consecutive interactions, typically consisting of the following: (a) ligand–receptor interactions, (b) intracellular signal transduction cascades between receptors and transcription factors and (c) transcription factors and targeted gene interactions. These Pathway Maps comprehensively cover human, mouse and rat canonical signalling and metabolism. In this analysis, the significance of the overlap (enrichment) was defined by P -values obtained from a hypergeometric distribution using the following formula (1): where: N =the total number of genes covered by the whole ontology R =the number of items in an input list (organ-enriched genes, sex-specific or development-dependent cluster of genes) n =the number of genes associated with a particular category from the ontology r =the number of objects in an input list (organ-enriched genes, sex-specific cluster or development-dependent cluster) intersecting with genes from a particular ontology category. For each set of organ-enriched genes, sex-specific cluster or development-dependent cluster, each list of up- and downregulated genes was associated with a quantitatively ranked list of ontology terms. This procedure summarized characteristics of the genes at a systems biology level. Significantly enriched ontology terms were those with an enrichment P -value 0.05. Alternative polyadenylation expression events To identify differentially expressed APA events, we first selected all the isoforms of an AceView gene model that have identical 5′ UTR and coding region. We then calculated the expression proportion P for the major isoform (2): Where a and b represented the two isoforms with an APA event, with a being the major isoform; FPKM was estimated by the Tophat–Cufflinks pipeline. Differential expression was tested by ANOVA and post-hoc multiple comparisons. A P close to one indicates a differential expression pattern of the two isoforms. Co-expression-based function prediction We identified genes with similar profile of expression across all organs and stages. Once these equivalence classes were set, we used GO annotation to propose a function for unannotated genes. Note that this procedure would not be limited to AceView-only genes but would apply to all genes and many RefSeq genes could be assigned proposed functions in the same way. We processed GO terms and expression profile data in two steps. As recommended by GO, expression pattern could only be used in some terms of biological processes, such as specific developmental stages in specific organs and process of stress response. Thus, we first set to identify GO terms whose members showed highly correlated expression profiles. By using the Wilcoxon–Mann–Whitney test (FDR<0.001), we identified bioprocesses for which the function of their members may be predictable by the expression profiles in this study. The alternative hypothesis was that the Pearson correlation coefficients (PCCs) of transcripts within the same GO term were not equal to that of all the PCCs of all the transcripts in the expression table. Then, for each unannotated AceView-only gene and a GO term, the maximum likelihood ratio was defined as (3): where LR is the maximum likelihood ratio; c is the maximum PCC between a transcript and T , which represents all the genes annotated within a given GO term. Rat RNA-Seq transcriptomic BodyMap database To facilitate community-wide use of this unique RNA-Seq data set, we created a web-based, open-access, user-friendly rat BodyMap database ( http://pgx.fudan.edu.cn/ratbodymap/index.html ). The database entries were linked to many other widely used databases, including AceView, GenBank, Entrez, Ensembl, RGD, UniProt, GO and Kyoto Encyclopedia of Genes and Genomes. Each gene with predefined expression features discussed above can be easily explored in the database. Users can query specific genes by using simple or complex search terms and can restrict the results to specific portions of the data set. For example, users can perform a query by entering an Entrez ID or gene symbol in the search box; selecting a region on the chromosome map or entering a specific chromosome region in search box; uploading user’s own DNA sequences for BLAST homology search; or just selecting items in the Browse page to view specific data. Our transcriptomic data can be visualized intuitively in various plots based on many different comparisons as needed. Accession codes: The Rat RNA-Seq BodyMap data set has been deposited in NCBI Gene Expression Omnibus (GEO) under accession code GSE53960 . How to cite this article: Yu, Y. et al . A rat RNA-Seq transcriptomic BodyMap across 11 organs and 4 developmental stages. Nat. Commun. 5:3230 doi: 10.1038/ncomms4230 (2014).